Actin–microtubule coordination at growing microtubule ends To power dynamic processes in cells, the actin and microtubule cytoskeletons organize into complex structures. Although it is known that cytoskeletal coordination is vital for cell function, the mechanisms by which cross-linking proteins coordinate actin and microtubule activities remain poorly understood. In particular, it is unknown how the distinct mechanical properties of different actin architectures modulate the outcome of actin–microtubule interactions. To address this question, we engineered the protein TipAct, which links growing microtubule ends via end-binding proteins to actin filaments. We show that growing microtubules can be captured and guided by stiff actin bundles, leading to global actin–microtubule alignment. Conversely, growing microtubule ends can transport, stretch and bundle individual actin filaments, thereby globally defining actin filament organization. Our results provide a physical basis to understand actin–microtubule cross-talk, and reveal that a simple cross-linker can enable a mechanical feedback between actin and microtubule organization that is relevant to diverse biological contexts. Eukaryotic cellular life critically relies on cell division, growth and migration, all highly dynamic processes that are organized and powered by the microtubule and actin cytoskeletons. Although it is now clear that these two cytoskeletal systems must be coordinated [1] , it remains unclear how the activity of actin–microtubule cross-linkers enables their functional co-organization in different cellular contexts. In particular, it is unknown how cross-linker-mediated cytoskeletal cross-talk is influenced by the diversity of filamentous actin (F-actin) architectures found in cells (that is, free, cross-linked and bundled), whose distinct mechanical properties are likely to impact the outcome of their encounters with growing microtubules. An important instance of actin–microtubule coordination in cells consists in guidance of microtubule growth by bundles of F-actin [1] . This occurs in migratory cells, where growing microtubule ends are targeted towards focal adhesions at the ends of stress fibres to regulate their turnover [2] , [3] , [4] and ensure motility [2] , and in extending axons, where microtubules that polymerize inside filopodia at the front of the growth cone consolidate the direction of growth [5] , [6] , [7] . Essential players in these processes are the spectraplakins [8] , such as the microtubule–actin cross-linking factor (MACF) [9] , [10] , multivalent proteins capable of both physically cross-linking F-actin and microtubules [2] , [6] , [7] , [8] , [9] , [10] , [11] , [12] , and transiently concentrating at growing microtubule ends by associating with end-binding (EB) proteins [6] , [12] , putting them in the class of plus-end tracking proteins (+TIPs [13] ). Other actin–microtubule cross-linking systems involving +TIP activity include the closely related GAS2-like family of proteins [14] , [15] , [16] and the Kar9-Bim1-Myo2 system of Saccharomyces cerevisiae [17] , [18] . Here, with the use of a minimal model system reconstituted from purified proteins, we elucidate how linking growing microtubule ends to F-actin structures can help direct cytoskeletal organization. To establish actin–microtubule interactions in vitro , we engineered a model actin-binding, microtubule plus-end tracking protein that we call TipAct. This simple cross-linking system recapitulates the in vivo ability of stiff actin bundles to capture and guide microtubule growth [2] , [3] , [4] , [5] , which turns out to be highly dependent on their encounter angle and the concentration of cross-linking protein both at the microtubule tip and the lattice. In a different context, however, the same cross-linking system enables growing microtubules to pull, stretch and bundle single actin filaments, and thereby globally dictate their spatial organization. We conclude that, independently of biochemical regulation, a variety of cytoskeletal organizations can arise from the interplay between a simple cross-linker and the relative mechanical properties of F-actin and microtubule structures. TipAct links microtubule growing ends to actin filaments We generated a minimal version of the F-actin binding +TIP MACF (also known as ACF7 in mammals [2] and short-stop/shot in Drosophila [11] ). Our green fluorescent protein (GFP)–TipAct construct ( Fig. 1a ; Supplementary Fig. 1a ) contains an N-terminal GFP-tag followed by an F-actin-binding domain consisting of tandem calponin-homology (CH) domains [9] , [11] , and an C-terminal region containing an SxIP motif to bind EB proteins [6] , [12] , [19] , and thus act as a microtubule tip localization signal (MtLS) [19] . We replaced the plakin domain and spectrin-repeat rod that separate these regions [8] (and may mediate dimerization [9] ) in MACF with the coiled-coil linker of cortexillin I, which induces parallel dimerization [20] . Despite its much simpler domain architecture, when transiently expressed in living cells, GFP–TipAct localized to the growing ends of microtubules and to F-actin structures in the periphery of the cell, in a similar fashion as full-length MACF/Shot do in vivo [6] , [7] , [9] , [10] , [12] , [21] , [22] ( Supplementary Fig. 1b,c ; Supplementary Information ). 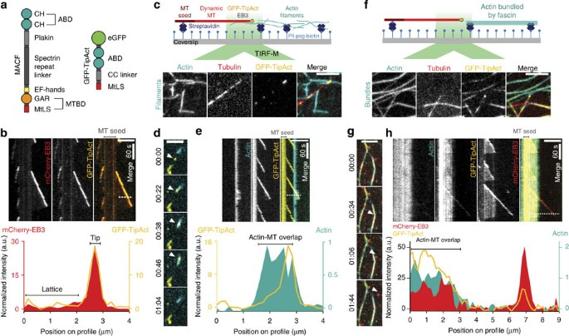Figure 1: GFP–TipAct localizes to growing microtubule ends via EB3 where it interacts with actin filaments, and also guides microtubule growth along actin bundles. (a) Domain structures of full-length MACF and GFP–TipAct. (b) Kymograph of microtubule growth with mCherry–EB3 and GFP–TipAct (top,Supplementary Movie 1). Fluorescence intensity along the dashed line on the kymograph (bottom). Experimental setups where growing microtubules interact with actin filaments (c) (top), or actin bundles (f) (top), via EB3 and TipAct. Montages showing the representative localization of GFP–TipAct in these experiments (c,f) (bottom). (d) Time series of an experiment as inc(top). Arrowheads show a microtubule growing plus-end that interacts with an actin filament (Supplementary Movie 2). (e) (top), kymograph of the microtubule ind. (e) (bottom), fluorescence intensity along the dashed line on the kymograph. (g) Time series of an experiment as inf(top). (h) (top), kymograph of the microtubule growing along an actin bundle, indicated by arrowheads ing(Supplementary Movie 3). (h) (bottom), fluorescence intensity along the dashed line on the kymograph. Inb,eandh, the location of the microtubule seed is indicated above the merge pane. The GFP–TipAct and mCherry–EB3 intensities were normalized by their mean values at the microtubule lattice, and the actin intensity by its mean value (when applicable). Composition inb,candd: 16 μM tubulin, 100 nM EB3 and 50 nM GFP–TipAct forn=5 experiments; infandg: 27 μM tubulin, 100 nM EB3, 50 nM GFP–TipAct and 500 nM fascin, forn=8 experiments. Scale bars, 5 μm; time, min:s. ABD, actin-binding domain; MT, microtubule; MtLS, microtubule tip localization signal; MTBD, microtubule-binding domain; CC, coiled-coil. Figure 1: GFP–TipAct localizes to growing microtubule ends via EB3 where it interacts with actin filaments, and also guides microtubule growth along actin bundles. ( a ) Domain structures of full-length MACF and GFP–TipAct. ( b ) Kymograph of microtubule growth with mCherry–EB3 and GFP–TipAct (top, Supplementary Movie 1 ). Fluorescence intensity along the dashed line on the kymograph (bottom). Experimental setups where growing microtubules interact with actin filaments ( c ) (top), or actin bundles ( f ) (top), via EB3 and TipAct. Montages showing the representative localization of GFP–TipAct in these experiments ( c , f ) (bottom). ( d ) Time series of an experiment as in c (top). Arrowheads show a microtubule growing plus-end that interacts with an actin filament ( Supplementary Movie 2 ). ( e ) (top), kymograph of the microtubule in d . ( e ) (bottom), fluorescence intensity along the dashed line on the kymograph. ( g ) Time series of an experiment as in f (top). ( h ) (top), kymograph of the microtubule growing along an actin bundle, indicated by arrowheads in g ( Supplementary Movie 3 ). ( h ) (bottom), fluorescence intensity along the dashed line on the kymograph. In b , e and h , the location of the microtubule seed is indicated above the merge pane. The GFP–TipAct and mCherry–EB3 intensities were normalized by their mean values at the microtubule lattice, and the actin intensity by its mean value (when applicable). Composition in b , c and d : 16 μM tubulin, 100 nM EB3 and 50 nM GFP–TipAct for n =5 experiments; in f and g : 27 μM tubulin, 100 nM EB3, 50 nM GFP–TipAct and 500 nM fascin, for n =8 experiments. Scale bars, 5 μm; time, min:s. ABD, actin-binding domain; MT, microtubule; MtLS, microtubule tip localization signal; MTBD, microtubule-binding domain; CC, coiled-coil. Full size image To test the +TIP activity of TipAct in vitro , we polymerized microtubules from GMPCPP-stabilized microtubule seeds immobilized on a microscope coverslip, in the presence of GFP–TipAct and mCherry–EB3 (EB protein family member 3), and imaged the proteins by total internal reflection fluorescence microscopy. GFP–TipAct localized to growing microtubule ends only when EB3 was present ( Fig. 1b ; Supplementary Fig. 2a ; Supplementary Movie 1 ). We did not observe lagging of TipAct’s plus-end intensity behind that of EB3 ( Fig. 1b , bottom), in contrast to MACF/Shot’s behaviour in vivo [6] , [12] , suggesting that other protein domains or interactions with F-actin may be required for this effect. Fluorescence recovery after photobleaching (FRAP) experiments revealed that both EB3 and TipAct exchange quickly at microtubule tips, k off ~2–3 s −1 ( Supplementary Fig. 3b,c ; Supplementary Information ). Finally, TipAct did not alter the parameters of microtubule dynamic instability relative to the addition of EB3 alone ( Supplementary Table 1 ). We thus conclude that on freely growing microtubules, TipAct behaves as an EB-dependent plus-end tracker with no added effect on microtubule dynamics. We then tested the interaction of TipAct with F-actin, and found that in the conditions of our in vitro assays (that is, [GFP–TipAct]~25–50 nM), GFP–TipAct did not detectably bind actin filaments on its own ( Fig. 1c , bottom). This can be explained by its low affinity for F-actin ( K d ~5 μM, Supplementary Fig. 4a ), which we measured via co-sedimentation assays, and is consistent with the dissociation constants of tandem CH actin-binding domains (ABDs) ( K d ~5–25 μM) typically reported in the literature [23] . Note, however, that this observation is at odds with previously reported values of MACF/Shot’s affinity for F-actin [11] , [22] , in which K d ’s in the order of 22–350 nM were estimated. Although we did not rule out that low affinity of GFP–TipAct for F-actin stems from steric hindrance by the enhanced GFP (eGFP) tag, we were careful to place spacers between all its functional domains ( Supplementary Fig. 1a ). A medium-to-low affinity for F-actin would be, however, more consistent with MACF/Shot’s predominant localization at microtubule tips and specific actin structures at the periphery of cells [6] , [7] , [9] , [10] , [12] , [21] , [22] , which we found well mimicked by our GFP–TipAct construct ( Supplementary Fig. 1b,c ). Despite the low affinity of TipAct for actin filaments, its locally enhanced concentration at the growing ends of microtubules could clearly lead to the binding of actin filaments, which was evidenced by a cessation in actin filament fluctuations at the point of capture by a growing microtubule ( Fig. 1d ; Supplementary Movie 2 ). This suggests that collective effects can enable an otherwise weak actin-binder to link the microtubule tip to F-actin. Such an effect could be essential for the in vivo activity of actin–microtubule cross-linking +TIPs, such as MACF/Shot or the GAS2-like family of proteins, allowing cells to control where microtubule cross-talk with single actin filaments takes place, that is, at growing microtubule ends, while avoiding cross-linking elsewhere. TipAct guides microtubule growth along actin bundles In stark contrast to the microtubule-dependent interactions with single actin filaments, we observed that GFP–TipAct stably and independently associated with actin bundles ( Fig. 1f bottom, Supplementary Fig. 2b ). A binding preference for bundles over single actin filaments has also been reported for Dystrophin [24] , a closely related protein to MACF/Shot with a homologous tandem CH ABD [8] . This property could help explain why MACF/Shot decorate specific pools of F-actin in cells [6] , [7] , [9] , [10] , [12] , [21] , [22] . TipAct’s stable association with actin bundles was sufficient to force microtubule growth to proceed in tight association with such bundles (an effect we call ‘zippering’; Fig. 1g ; Supplementary Movie 3 ). This was the result of TipAct-mediated localization of EB3 at actin bundles ( Supplementary Fig. 2b top), which was further enhanced in regions of microtubule–actin overlap ( Fig. 1h ; Supplementary Fig. 2b bottom). Similar effects on EB1 localization and actin–microtubule co-alignment have been recently reported for members of the GAS2-like family of proteins in vivo [15] , and could help explain the observed enhancement of MACF/Shot and EB1 localization along microtubules in actin-rich regions in cells [10] , [12] . It is plausible that in vivo such a mechanism acts in synergy with the establishment of actin–microtubule linkages mediated by MACF/Shot’s microtubule lattice-binding domain [6] , [8] ( Fig. 1a ), which is the most heavily regulated portion of these molecules [21] , [25] , [26] . Note that we never observed guidance of microtubule growth by actin bundles, nor enhanced mCherry–EB3 localization at actin bundles when we replaced TipAct for a similar protein construct lacking the ABD altogether ( Supplementary Fig. 2c ; Supplementary Movie 4 ). To test whether the establishment of an actin–microtubule connection would affect EB3 and TipAct’s turnover rates, we performed FRAP experiments on free and actin-bound microtubule tips, as well as on free and microtubule-bound actin bundles, and tracked the fluorescence recovery of mCherry–EB3 and GFP–TipAct for all cases ( Supplementary Fig. 3 ; Supplementary Information ). Consistent with previously reported values [27] , mCherry–EB3 and GPF–TipAct both exchanged quickly at free microtubule growing ends ( k off ~2–3 s −1 ; Supplementary Fig. 3b,c ). In the case of actin-bound microtubule tips, however, we found that a fraction of these proteins exchanged approximately three to five times slower ( Supplementary Fig. 3b,c ). In addition, the transition rate from a tip-like to a lattice-like binding profile was reduced twofold (resulting in longer plus-end intensity profiles, given that microtubule growth rates remained the same; Supplementary Fig. 3c ), and the steady-state microtubule lattice-intensity of both mCherry–EB3 and GFP–TipAct increased ( Supplementary Fig. 3b ). On the other hand, we found that GFP–TipAct stably associated with actin bundles (both free and microtubule bound) showing no recovery on the timescale of observation (~14 s). However, mCherry–EB3 was mobile in both cases ( Supplementary Fig. 3f ), although we found that a fraction of the protein recovered approximately three times slower in the presence of actin–microtubule overlaps ( Supplementary Fig. 3g ). These experiments reveal two important things: first, that EB3 and TipAct do not form a stable complex in solution, but rather dissociate on a timescale (~3 s) that is slower than their dwell-time at microtubule growing ends (~0.3–0.5 s), but faster than the dwell-times of TipAct at actin bundles (>14 s), and of EB3 at the microtubule lattice in regions of actin–microtubule overlap (~10 s). Second, that actin–microtubule linkages can be stabilized by the steady localization of TipAct at actin bundles, which leads to a reduced off-rate of EB3 in regions of actin–microtubule overlap, effectively resulting in enhanced steady-state microtubule tip and lattice intensities of both proteins. Supplementary Fig. 3d,h show schematics of the interpretation of the FRAP experiments, and the different reactions with which we associate the rates ( Supplementary Fig. 3c,g ) obtained from fits to the recovery curves ( Supplementary Information ). Actin bundles can capture and redirect microtubule growth Given that TipAct allows actin bundles to guide microtubule growth, we wondered whether this interaction could lead to the efficient capture and redirection of growing microtubule ends. For this purpose, we characterized encounters between growing microtubules and actin bundles, and classified their outcome into four categories [28] : catastrophe, cross-over, deflection and zippering ( Fig. 2a ), whose probability we analysed as a function of microtubule length L and intersection angle θ between the microtubule and the actin bundle at the point of first contact. Without TipAct, microtubule ends could be deflected by collisions with the actin bundles, leading to smooth bending of the microtubules as they continued to grow ( Fig. 2b ; Supplementary Movie 5 ). This effect was dominant at shallow angles (<5°), was rare above 25° ( Fig. 2c ) and its probability weakly increased with microtubule length ( Fig. 2f , top). Catastrophes were observed at all angles, but more often for short microtubules ( Fig. 2f , top). 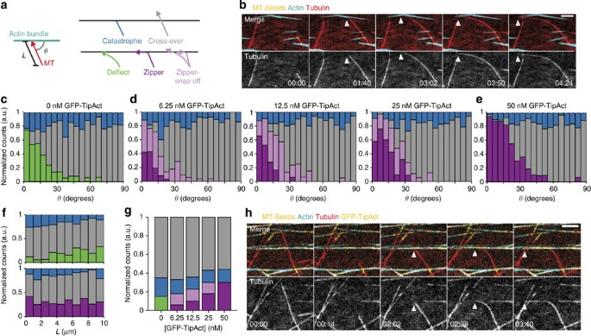Figure 2: GFP–TipAct captures and redirects microtubule growth along actin bundles. (a) Classification of the interaction outcome between growing microtubule plus-ends and actin bundles, and how the intersection angleθand microtubule lengthLwere defined. (b) Time series of a microtubule grown without GFP–TipAct whose plus-end is mechanically deflected by an actin bundle (Supplementary Movie 5). Analysis of the probability of each interaction outcome as defined ina, as a function ofθ, both without (c) and with increasing concentrations of GFP–TipAct (d,e). (f) Analysis of the probability of each interaction outcome as a function ofLwith (bottom) or without (top) 50 nM GFP–TipAct. (g) Comparison of the compound probability of each outcome for all the concentrations of GFP–TipAct used. For each of the following conditions: 0, 6.25, 12.5, 25 and 50 nM GFP–TipAct,n=708, 459, 421, 443 and 914 interactions were analysed, respectively. (h) Time series of a microtubule grown with GFP–TipAct that zippers onto an actin bundle as it grows (Supplementary Movie 6). Composition: 25 μM tubulin, 100 nM EB3 and 500 nM fascin forn=6 experiments with (h) andn=9 experiments without (b) 50 nM GFP–TipAct. Inbandh, white arrowheads indicate the growing plus-ends of the microtubules. Scale bars, 10 μm; time, min:s. Figure 2: GFP–TipAct captures and redirects microtubule growth along actin bundles. ( a ) Classification of the interaction outcome between growing microtubule plus-ends and actin bundles, and how the intersection angle θ and microtubule length L were defined. ( b ) Time series of a microtubule grown without GFP–TipAct whose plus-end is mechanically deflected by an actin bundle ( Supplementary Movie 5 ). Analysis of the probability of each interaction outcome as defined in a , as a function of θ , both without ( c ) and with increasing concentrations of GFP–TipAct ( d , e ). ( f ) Analysis of the probability of each interaction outcome as a function of L with (bottom) or without (top) 50 nM GFP–TipAct. ( g ) Comparison of the compound probability of each outcome for all the concentrations of GFP–TipAct used. For each of the following conditions: 0, 6.25, 12.5, 25 and 50 nM GFP–TipAct, n =708, 459, 421, 443 and 914 interactions were analysed, respectively. ( h ) Time series of a microtubule grown with GFP–TipAct that zippers onto an actin bundle as it grows ( Supplementary Movie 6 ). Composition: 25 μM tubulin, 100 nM EB3 and 500 nM fascin for n =6 experiments with ( h ) and n =9 experiments without ( b ) 50 nM GFP–TipAct. In b and h , white arrowheads indicate the growing plus-ends of the microtubules. Scale bars, 10 μm; time, min:s. Full size image With TipAct, capture of microtubule ends occurred over a similar range of angles ( Fig. 2e ), but was, however, followed by zippered growth along the actin bundles. This could result in sharp bends of the microtubule lattice near the point of first contact ( Fig. 2h ; Supplementary Movie 6 ), reminiscent of recent observations of microtubule guidance by actin stress fibres in patterned cells, in which microtubules were observed to sustain sharp deformations [29] . Capture of microtubule ends by TipAct reduced the probability of microtubule catastrophe-induced by collisions [30] at small encounter angles ( Fig. 2e ), and made capture insensitive to microtubule length ( Fig. 2f , bottom). Similar observations of microtubule capture and guidance have been recently reported using EB1–kinesin complexes in vitro [31] , [32] . To test the contributions of microtubule tip and lattice to the capture and guidance mechanism of TipAct, we performed further experiments with decreasing amounts of TipAct while keeping EB3 constant. We found that while the angle dependency for microtubule capture remained approximately the same; reducing the concentration of GFP–TipAct resulted in an increasing fraction of zippering microtubules that eventually snapped off their actin tracks ( Fig. 2d ). This was true for both steep ( Supplementary Fig. 5a ; Supplementary Movie 7 ) and shallow ( Supplementary Fig. 5b ) encounter angles. Furthermore, at the lowest concentration of GFP–TipAct used, we found that a large fraction of microtubules interacted with the actin bundles solely via their growing tips ( Supplementary Fig. 5c ), resulting in a guidance mechanism that closely resembled that of deflection ( Fig. 2b ) when TipAct was fully absent. These observations indicate that the bending energy involved in redirecting a microtubule can only be overcome by physically linking its lattice to the actin bundle, effectively leading to increased capture and alignment efficiency ( Fig. 2g ). Although the microtubule tip plays a key role in the initial capture event (we never observed a microtubule aligning with an actin bundle that it had initially crossed-over), decreasing the amount of TipAct revealed that when the density of cross-linkers at the actin–microtubule overlap is not high enough, and given that EB3 does exchange ( Supplementary Fig. 3 ), microtubules will be more likely to detach from their actin tracks. Arrays of actin bundles globally organize microtubule growth Given that both mechanical effects and physical cross-linking by TipAct can redirect microtubule growth, albeit with different efficiency, we wondered to what extent they would allow a well-defined F-actin architecture to globally organize microtubule growth. To this end, we generated sparse arrays of actin bundles interspersed with randomly oriented microtubule seeds from which microtubules were polymerized in quasi two-dimensional confinement [33] . Growth was allowed to proceed for ~1 h, with ( Fig. 3a ) and without ( Fig. 3b ) GFP–TipAct, in conditions where the average microtubule length continuously increased ( Supplementary Fig. 6 ; Supplementary Information ). In both cases, histograms of microtubule orientation angle θ MT gradually developed a peak centred about the mean F-actin angle 〈θ ACTIN 〉 ( Fig. 3c ), although with TipAct the final peak appeared narrower, and the microtubules better co-aligned with the actin bundles ( Fig. 3a,b ). 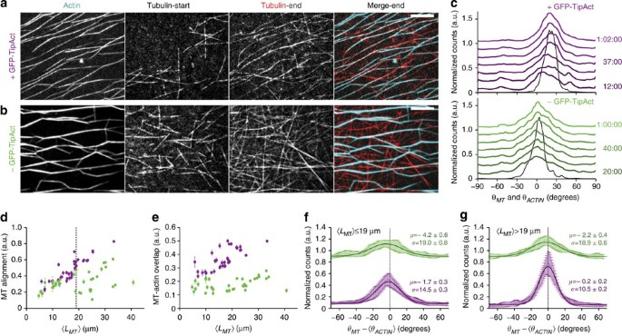Figure 3: GFP–TipAct allows linear arrays of actin bundles to stably and efficiently template microtubule organization. Early (t=0) and late (t~40–50 min) time points of microtubule growth within linear arrays of actin bundles with (a), and without (b) GFP–TipAct. (c) Evolution of the distributions of microtubule orientation angleθMT, for the experiments inaandb, respectively. Colour gradients indicate the time evolution of the distribution. Each curve is shifted 0.17 a.u. relative to the previous one. Black curves show the time-averaged distribution of actin-bundle orientation angleθACTIN. Evolution of microtubule alignment (d), and microtubule–actin overlap (e), as functions of〈LMT〉. Error bars are s.d. The gray-dashed line at〈LMT〉=19 μm indindicates where the trends diverge. Normalized histograms of the difference between microtubule and mean F-actin orientation angle〈θACTIN〉, for short (f), and long (g), microtubules as defined ind. Data are the average ofn=6/9 experiments, comprising 17/9 histograms for long microtubules, and 18/11 histograms for short microtubules, with/without GFP–TipAct, respectively. Error bars are s.d. Dark green and purple lines and insets show fits to equation (1) (see Methods). Data and fits without GFP–TipAct are shifted up 0.8 a.u. Composition of the experiments: 27 μM tubulin, 100 nM EB3 and 500 nM fascin; with (a) and without (b) 50 nM GFP–TipAct. Scale bars, 10 μm; time, h:min:s. MT, microtubule. Figure 3: GFP–TipAct allows linear arrays of actin bundles to stably and efficiently template microtubule organization. Early ( t =0) and late ( t ~40–50 min) time points of microtubule growth within linear arrays of actin bundles with ( a ), and without ( b ) GFP–TipAct. ( c ) Evolution of the distributions of microtubule orientation angle θ MT , for the experiments in a and b , respectively. Colour gradients indicate the time evolution of the distribution. Each curve is shifted 0.17 a.u. relative to the previous one. Black curves show the time-averaged distribution of actin-bundle orientation angle θ ACTIN . Evolution of microtubule alignment ( d ), and microtubule–actin overlap ( e ), as functions of 〈L MT 〉 . Error bars are s.d. The gray-dashed line at 〈L MT 〉 =19 μm in d indicates where the trends diverge. Normalized histograms of the difference between microtubule and mean F-actin orientation angle 〈θ ACTIN 〉 , for short ( f ), and long ( g ), microtubules as defined in d . Data are the average of n =6/9 experiments, comprising 17/9 histograms for long microtubules, and 18/11 histograms for short microtubules, with/without GFP–TipAct, respectively. Error bars are s.d. Dark green and purple lines and insets show fits to equation (1) (see Methods). Data and fits without GFP–TipAct are shifted up 0.8 a.u. Composition of the experiments: 27 μM tubulin, 100 nM EB3 and 500 nM fascin; with ( a ) and without ( b ) 50 nM GFP–TipAct. Scale bars, 10 μm; time, h:min:s. MT, microtubule. Full size image To better quantify this difference in organization efficiency, we calculated the degree of microtubule alignment ( Supplementary Information ) for several such experiments as a function of the average microtubule length ( 〈L MT 〉 ), which we estimated from the fraction of the field of view covered by microtubules ( Supplementary Fig. 7 ; Supplementary Information ). For short microtubules ( 〈L MT 〉 ≤19 μm), alignment increased linearly with 〈L MT 〉 , both with and without TipAct ( Fig. 3d ). However, for long microtubules ( 〈L MT 〉 >19 μm) these trends diverged: with TipAct microtubules became increasingly aligned, whereas without TipAct there was no discernible trend in alignment with increasing length. As expected, in the presence of TipAct, increased microtubule alignment coincided with increased overlap with the actin bundles as a result of zippering ( Fig. 3e ). Thus, although purely mechanical effects can under certain conditions organize microtubule growth ( Fig. 2b,c ), lack of (sufficient) anchoring to the actin bundles eventually makes microtubules susceptible to lose their tracks ( Fig. 2d ; Supplementary Fig. 5 ), which is especially true if the actin bundles are sparse [33] . We anticipate that in a three-dimensional cellular situation, such ‘escapes’ would be even more common. On average, microtubule zippering via EB3 and TipAct resulted in sharper microtubule orientation distributions better centred about the average actin bundle orientation 〈θ ACTIN 〉 , both for short ( 〈L MT 〉 ≤19 μm, Fig. 3f ), and long ( 〈L MT 〉 >19 μm, Fig. 3g ) microtubules. Such efficiency in actin–microtubule co-alignment may account for the in vivo observation that the activity of cross-linkers such as MACF/Shot is necessary to establish well-ordered arrays of parallel microtubules oriented towards the cell edge [2] , [10] . Given that growth proceeds tightly along the actin bundle, potentially protecting the microtubule tip from the many obstacles ubiquitous to the crowded interior of the cell, we speculate that physically linking the elongating microtubule lattice to the actin bundles is likely to be one of the most efficient ways to target microtubule growth to particular sites in the cell, such as focal adhesions at the end of actin stress-fibres [2] , [3] , [4] , or to the ends of filopodia [5] , [6] , [7] . Growing microtubules can dictate actin filament organization Having shown how arrays of actin bundles can impose their organization on growing microtubules, we wondered whether microtubules could, conversely, impose their organization on actin filaments. Indeed, transient interactions between microtubule growing ends and actin filaments through EB3 and TipAct ( Fig. 1d,e ) were sufficient to allow microtubules to capture and transport freely diffusible actin filaments ( Fig. 4a ; Supplementary Movie 8 ), and to pull and stretch actin filaments that were partially attached to the coverslip ( Fig. 4b ; Supplementary Movie 9 ), independent of actin filament polarity ( Supplementary Fig. 8a ; Supplementary Movie 10 ). Given the low affinity of GFP–TipAct for actin filaments ( Supplementary Fig. 4a ), these force-generating interactions presumably stem from collective binding events taking place at the microtubule tip, in our eyes analogous to the way kinetochore components track depolymerizing microtubules [34] . A similar force-generation mechanism is at play in recent reports of microtubule growing ends pulling membrane tubes via +TIPs anchored at the endoplasmic reticulum [35] . 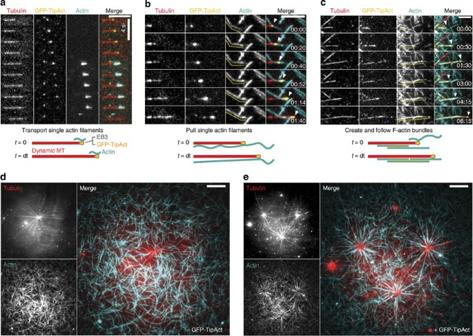Figure 4: GFP–TipAct allows growing microtubules to transport, pull and bundle actin filaments, globally dictating F-actin organization. (a) Time series of a growing microtubule end that transports a short actin filament (Supplementary Movie 8). Schematic of this effect (bottom). (b) Time series of a growing microtubule that aligns and then pulls on an actin filament (Supplementary Movie 9). The dashed yellow line in the actin pane shows the contour changes of the actin filament. Arrowheads in the merge pane show the microtubule plus-end. Schematic of this effect (bottom). (c) Time series of a growing microtubule that captures actin filaments and forms a bundle, which then guides the growth of another microtubule (Supplementary Movie 11). The dashed yellow line in the actin pane shows the formation of the bundle. White arrowheads and arrows in the merge pane show the growing plus-ends of these two microtubules. Schematic of this effect (bottom). Steady-state F-actin organization in the vicinity of a radial array of dynamic microtubules, with (e), and without (d) GFP–TipAct. Composition inaandb: 16 μM tubulin, 100 nM EB3 and 50 nM GFP–TipAct forn=8 and 9 experiments, respectively; inc: 20 μM tubulin, 100 nM EB3 and 25 nM GFP–TipAct forn=10 experiments; indande: 20 μM tubulin, 100 nM EB3, with (e) and without (d) 200 nM GFP–TipAct forn=20 and 5 experiments, respectively. Scale bars, 5 μm (a–c); 10 μm (d,e); time, min:s. MT, microtubule. Figure 4: GFP–TipAct allows growing microtubules to transport, pull and bundle actin filaments, globally dictating F-actin organization. ( a ) Time series of a growing microtubule end that transports a short actin filament ( Supplementary Movie 8 ). Schematic of this effect (bottom). ( b ) Time series of a growing microtubule that aligns and then pulls on an actin filament ( Supplementary Movie 9 ). The dashed yellow line in the actin pane shows the contour changes of the actin filament. Arrowheads in the merge pane show the microtubule plus-end. Schematic of this effect (bottom). ( c ) Time series of a growing microtubule that captures actin filaments and forms a bundle, which then guides the growth of another microtubule ( Supplementary Movie 11 ). The dashed yellow line in the actin pane shows the formation of the bundle. White arrowheads and arrows in the merge pane show the growing plus-ends of these two microtubules. Schematic of this effect (bottom). Steady-state F-actin organization in the vicinity of a radial array of dynamic microtubules, with ( e ), and without ( d ) GFP–TipAct. Composition in a and b : 16 μM tubulin, 100 nM EB3 and 50 nM GFP–TipAct for n =8 and 9 experiments, respectively; in c : 20 μM tubulin, 100 nM EB3 and 25 nM GFP–TipAct for n =10 experiments; in d and e : 20 μM tubulin, 100 nM EB3, with ( e ) and without ( d ) 200 nM GFP–TipAct for n =20 and 5 experiments, respectively. Scale bars, 5 μm ( a – c ); 10 μm ( d , e ); time, min:s. MT, microtubule. Full size image When microtubules interacted simultaneously with many actin filaments, we observed that they could incorporate them into bundles that subsequently recruited GFP–TipAct and could thus act as guides for repeated rounds of microtubule growth ( Fig. 4c ; Supplementary Movie 11 ). Similar observations of composite actin–microtubule bundle formation have been reported for members of the closely related GAS2-like family of proteins in overexpression conditions [15] , [16] . Strikingly, in cases when the actin bundle was mobile, and its compliance comparable to that of the microtubule, we observed that both could deform as the microtubule polymerized ( Supplementary Fig. 8 ; Supplementary Movie 12 ). This observation is reminiscent of reports of microtubule-dependent reorganization of filopodia in cells [36] , and further supports the notion that mechanical effects strongly modulate the ability of physical cross-linkers to dictate actin–microtubule co-organization. Finally, to test whether these effects on single actin filaments ( Fig. 4a–c ) would allow microtubules to globally impose their organization on F-actin, we monitored the radial growth of microtubules nucleated by centrosomes immersed in an isotropic solution of actin filaments. Indeed, with GFP–TipAct, actin filaments in the vicinity of the microtubule array progressively adopted the radial organization ( Fig. 4e ; Supplementary Fig. 9 ; Supplementary Information ), while without it they largely ignored the microtubule array and remained free and randomly organized ( Fig. 4d ). Overall, our results reveal that the activity of a simple actin–microtubule cross-linking +TIP can establish a complex mechanical feedback between actin and microtubule organization. The affinity of TipAct is high for the ends of growing microtubules and actin bundles but low for actin filaments, which makes it possible to control the outcome of its cross-linking activity by defining the F-actin architecture and its rigidity relative to that of a microtubule. Our findings, although in the context of a highly simplified in vitro system, mirror observations reported in living cells, and highlight the physical component of the regulatory control that cells can exert on actin–microtubule co-organization in different contexts. All reagents were obtained from Sigma unless otherwise noted. Plasmid construction GFP–TipAct was designed to contain an N-terminal eGFP tag followed by the ABD and EB-binding domain (MtLS) of full-length human MACF1 (NCBI reference sequence: NP_036222.3), separated by the coiled-coiled linker of Cortexillin I [20] ( Supplementary Fig. 1a ). Using PCR-based strategies, we obtained the five necessary fragments: eGFP, ABD (first and second CH domains, corresponding to residues Asp74—Gly306 of full-length MACF1), Cortexillin I coiled-coiled linker (CC linker) and MtLS (corresponding to residues Glu5391—Arg5430 of full-length MACF1), from the following complementary DNA clones: pEGFP-C2 (Clontech, Takara Bio Europe, Saint-Germain-en-Laye, France), IMAGE clone 30414356, LIFESEQ5427393 (Open Biosystems, Thermo Fischer, Huntsville, AL, USA), full-length Cortexillin-I in pET-15b [20] and IMAGE clone 7476004. Each fragment was amplified using the primers indicated in Supplementary Table 2 . For protein purification, the amplified fragments were ligated into the bacterial expression vector: pET-28a (Novagen, Merck Millipore, Billerica, MA, USA), between Nde I and Bam HI sites. This procedure resulted in a vector expressing the construct eGFP–ABD–CC linker–EB-BD with an N-terminal thrombin-cleavable 6xHis tag for purification. For live-cell imaging experiments, the amplified fragments were ligated into the pEGFP-C2 vector (Clontech, Palo Alto, CA, USA) between the Nhe I and Bam HI sites. Protein isolation The E. coli strain T7-express (New England Biolabs, Ipswich, MA, USA) was used for expression of GFP–TipAct. Bacteria were grown at 37 °C in LB containing 50 μg ml −1 kanamycin. Protein expression was induced when cultures reached A 600 =0.8 by adding isopropyl β- D -1-thiogalactopyranoside to a final concentration of 0.4 mM, followed by further incubation at 20 °C overnight. The N-terminal 6xHis-tagged fusion proteins were affinity purified by immobilized metal-affinity chromatography on Ni-NTA agarose (Qiagen Benelux B.V., Venlo, Netherlands) at 4 °C using the gravity-flow method. Before cleavage of the 6xHis tag, proteins were diluted to a concentration of 5 mg ml −1 in gel filtration buffer (50 mM Na-phosphate pH 7, 400 mM NaCl, 2 mM MgCl 2 , 10% (v/v) glycerol and 5 mM β-mercaptoethanol) supplemented with 1 mM EDTA. Proteolytic cleavage was carried out overnight at room temperature (RT) using human thrombin at a concentration of 2.5 U mg −1 of protein. Uncleaved proteins were removed by running the cleavage reaction through the Ni-NTA agarose again. Cleaved proteins were concentrated with a 30-kDa MWCO centrifugal filter unit (Merck Millipore) and gel-filtered with an Äkta chromatography system (GE Healthcare Bio-Sciences AB, Uppsala, Sweden) through a Superdex-200 column (GE Healthcare) equilibrated in gel filtration buffer. The peak fractions were pooled and concentrated as above to a final concentration of 5 mg ml −1 , accompanied by a buffer exchange to MRB80-KGβ (MRB80: 80 mM Pipes, pH 6.8 set with KOH, 4 mM MgCl 2 and 1 mM EDTA, supplemented with 250 mM KCl, 10% (v/v) glycerol and 5 mM β-mercaptoethanol). Finally, the proteins were aliquoted, snap-frozen in liquid N 2 and stored at −80 °C. The homogeneity of the recombinant proteins was assessed by SDS–polyacrylamide gel electrophoresis (PAGE), and their concentration estimated from the optical absorbance in MRB80-KGβ buffer at a wavelength of 280 nm with an extinction coefficient of 59,820 M −1 cm −1 (estimated from the amino-acid sequence). To obtain uncleaved 6xHis-GFP–TipAct, the purification protocol was stopped after elution from the first Ni-NTA step, the protein was concentrated as above to a final concentration of 5 mg ml −1 , accompanied by a buffer exchange to MRB80-KGβ buffer, before snap-freezing and storage at −80 °C. Lyophilized porcine brain tubulins were obtained from Cytoskeleton (Denver, CO, USA), resuspended at 50–100 μM in MRB80, snap-frozen and stored at −80 °C until use [33] . G-Actin was purified from rabbit skeletal muscle acetone powder [37] , [38] and kept at 4 °C for daily use, or at −80 °C for long-term storage [33] . Alexa Fluor 647 and 594 succinimidyl ester dyes (Molecular Probes, Life Technologies, Carlsbad, CA, USA) were used to produce labelled G-actin [37] . Glutathione S -transferase-tagged recombinant human fascin (generous gift from Dyche Mullins, UCSF, San Francisco, CA, USA) was expressed and purified via affinity chromatography on a glutathione-containing matrix, and the glutathione S -transferase-tag removed via the PreScission protease sytem according to the manufacturer’s protocols (GE Healthcare) [33] , [37] . 6xHis-tagged recombinant human EB3, GFP–EB3, mCherry–EB3 and GFP–Tip (elsewhere called GFP-MACF43 (ref. 19 )) were expressed and purified with similar protocols as GFP–TipAct [19] , [39] , [40] . Centrosomes were purified with the generous help of Claude Celati (Institut Curie, Section Recherche, UMR144-CNRS, 75005 Paris, France), from human lymphoblastic KE37 cell lines. The homogeneity of all recombinant proteins used in this study was confirmed by SDS–PAGE ( Supplementary Fig. 4b ). Stabilized microtubule seeds and F-actin Stabilized microtubule seeds were prepared using the slowly hydrolysable GTP analogue guanylyl-(α,β)-methylene-diphosphonate (GMPCPP, Jena Biosciences, Jena, Germany) [33] . For the experiments with actin bundles or single filaments, phalloidin-stabilized F-actin was polymerized at a 1.0–1.5 μM final G-actin concentration, and for the experiments with centrosomes at 30 μM G-actin [33] . Co-sedimentation assays with GFP–TipAct and actin filaments G-actin (80 μM) was polymerized into F-actin for 1 h at RT in MRB80 containing 50 mM KCl and an equimolar amount of phalloidin. Samples of increasing F-actin concentration (0–50 μM) were incubated with 1 μM GFP–TipAct at RT for 1 h. Thereafter, bound and free fractions were separated by high-speed centrifugation at 149,000 g for 30 min at RT. Pellet and supernatant samples were brought to the same final volume and prepared for SDS–PAGE. The bound and free fractions of GFP–TipAct were estimated with the Gel Analyzer tool in FIJI [41] . The dissociation constant ( K d ) of GFP–TipAct for F-actin was estimated by fitting the data in Supplementary Fig. 4b to the equation: X bound =[ A ]/([ A ]+ K d ). Where X bound is the fraction of GFP–TipAct bound, and [ A ] the corresponding actin concentration. Preparation of flow cells for in vitro assays Glass coverslips (Menzel-Glässer, Braunschweig, Germany) were cleaned in base-piranha. Glass slides (Menzel-Glässer) were cleaned by sequential sonication in: 0.1% (v/v) Hellmanex, 100% acetone and 70% ethanol solutions in Milli-Q water, with 5-min rinses in Milli-Q water in between. Both glass coverslips and slides were stored at RT in a 0.1-M KOH solution until use [33] . Flow cells channels (~7–10 μl) were assembled by cutting ~2-mm-wide channels in a piece of Parafilm, which was sandwiched between clean glass slides and coverslips [33] . For the experiments with centrosomes, flow cells were assembled using silicon grease to both make 5–6 μl channels and to join glass the slide and coverslip together. Surface preparation for in vitro assays Biotinylated glass surfaces were obtained by sequentially incubating the flow cell channels with the following solutions: 0.2 mg ml −1 PLL-PEG-Biotin (PLL(20)-g[3.5]-PEG(2)/PEG(3.4)-Biotin, Susos AG, Dübendorf, Switzerland) for 30–45 min, 50–100 μg ml −1 streptavidin or neutravidin (Thermo Scientific Pierce Protein Biology Products, Rockford, IL, USA) for 10 min, 0.5 mg ml −1 κ-casein for 10 min and 1% (w/v) Pluronic F-127 for 10 min, all diluted in MRB80, with 50–100 μl rinses with MRB80 in between steps. Dynamic microtubules were nucleated from GMPCPP-stabilized microtubule seeds bound to biotinylated glass surfaces. ‘Landing’ of the seeds was aided by diluting them in MRB80 containing 0.1% (v/v) methyl cellulose. And any non-attached seeds were always rinsed with MRB80 before the actin filaments and/or the microtubule polymerization mix was added. For the experiments with linear arrays of fascin-bundled actin, we worked with special flow cells that had entry/exit holes on the glass-slide side from which all solutions where flowed [33] . Linear arrays of actin bundles were created in a sequence of steps: first, F-actin was flowed into the channels at the equivalent of ~1–2 μM G-actin concentration; second, a drop of 1.0% (v/v) methyl cellulose was placed at one end of the channel, and allowed to diffuse in for 5 min to induce F-actin bundling by depletion forces, push the bundles onto the coverslip surface and force the actin bundles to partially align [33] . Third, the channel was slowly rinsed with a 500-nM fascin and 0.1% (v/v) methyl cellulose solution in MRB80 to stabilize the actin bundles and remove excess methyl cellulose. To keep the bundles intact, fascin was kept at the same concentration in the channel for the rest of the experiment. For the experiments with centrosomes, flow cell channels were incubated for 8 min with a centrosome solution in MRB80 (pre-warmed to 37 °C for 30 min), which resulted in centrosomes non-specifically binding to the glass. Afterwards the channels were sequentially blocked with a 0.2 mg ml −1 PLL-PEG-Biotin solution for 8 min, followed by 0.5 mg ml −1 κ-casein solution for 5–10 min, all in MRB80. Microtubule end-tracking assays, with and without F-actin Once the flow cell channel surface was prepared with microtubule seeds (or centrosomes), and either fascin-bundled F-actin, single actin filaments or none, the microtubule polymerization mix was added. The core reaction mix consisted of: 0.5 mg ml −1 κ-casein, 0.1% (v/v) methyl cellulose, 50–75 mM KCl, 1 mM GTP and an oxygen scavenging system (4 mM dithiothreitol, 0.2 mg ml −1 catalase, 0.4 mg ml −1 glucose oxidase and 25–50 mM glucose) in MRB80. The tubulin concentration (always at a ratio of 1:15 labelled to unlabelled subunits) was varied depending on the experiment: for all the assays without actin it was kept at 16 μM, for the assays with linear arrays of actin bundles or with weakly bound actin filaments it was kept between 25–30 μM and for the experiments with centrosomes it was kept at 20 μM. Typically higher tubulin concentrations were used for the co-alignment experiments to obtain longer microtubules. The EB3 concentration (of either: EB3, GFP or mCherry-labelled EB3) was always kept at 100 nM, and the GFP–TipAct concentration was kept at 50 nM (unless otherwise noted). For the experiments with fascin-bundled F-actin, the microtubule polymerization reaction was supplemented with 500 nM fascin. For experiments with the actin-binding deficient GFP–Tip, its concentration was kept at 50 nM. For experiments with single actin filaments, F-actin was incorporated to the microtubule polymerization mix at what would be the equivalent of 100–200 nM G-actin concentration. For the experiments with centrosomes, the actin filaments were also directly incorporated into the microtubule polymerization mix, which consisted of the same core reaction mixture explained above plus 20 μM final tubulin concentration (1:15 labelled to unlabelled subunits), phalloidin-stabilized actin filaments equivalent to 0.7–1.0 μM G-actin concentration, 100 nM unlabelled EB3 and 200 nM GFP–TipAct. After mixing (before the addition of actin filaments for the experiments with centrosomes), the microtubule polymerization reaction mixture was clarified at 149,000 g for 5 min and immediately added to the flow cell channel, which was finally sealed either with wax or vacuum grease to avoid solvent evaporation while imaging. TIRF microscopy and FRAP Triple-colour TIRF microscopy and FRAP experiments were performed on an Nikon Eclipse Ti-E inverted microscope (Nikon Corporation, Tokyo, Japan) equipped with an Apo TIRF 100 × 1.49 N.A. oil objective, a motorized stage, Perfect Focus System, a motorized TIRF illuminator (Roper Scientific, Tucson, AZ, USA) and a QuantEM:512SC EMCCD camera (Photometrics, Roper Scientific). For excitation, we used a 561 nm (50 mW) Jive (Cobolt, Solna, Sweden) and a 488-nm (40 mW) Calypso (Cobolt) diode-pumped solid-state laser, and a 635-nm 28-mW Melles Griot laser (CVI Laser Optics & Melles Griot, Didam, Netherlands). For FRAP experiments, the microscope was equipped with a MAG Biosystems FRAP-3D system (Photometrics, Roper Scientific) that could either be used to do FRAP-on-the-fly (point FRAP) or region of interest FRAP experiments with diffraction-limited spots. Most of the imaging of dynamic microtubules was performed at 2 s per frame with 100–200 ms exposure time at 10–15% laser power, except for the experiments with centrosomes, which were imaged at 5 s per frame. FRAP experiments on mCherry–EB3 and GFP–TipAct at growing microtubule ends and actin bundles were performed at video rate (33 ms exposure time per frame), 10–15% laser power for imaging and 100% laser power for photobleaching. The sample temperature was controlled with the use of a home-built objective heater/cooler, and was varied depending on the desired range of microtubule lengths. For the experiments without actin, or with single actin filaments weakly bound to the coverslip, it was kept at 25±1 °C, for the assays with linear arrays of actin bundles it was kept between 32 and 34±1 °C and for the experiments with centrosomes the temperature was maintained at 30±1 °C. Image processing and data analysis All image processing and data analysis were performed using plugins for FIJI [41] or ImageJ [42] and custom-written programs in MATLAB (MathWorks Inc., Natick, MA, USA). Analysis of microtubule dynamic instability The parameters of microtubule dynamic instability ( Supplementary Table 1 ) were determined by analysing kymographs of microtubule growth produced using the reslice tool in FIJI [41] . Growth and shrink speeds were obtained from manual fits to the growth and shrinkage phases, and the average speeds weighted by the time the microtubules spent growing or shrinking at a given speed [43] . Catastrophe and rescue rates were obtained by dividing the total number of events by the total time microtubules spent growing or shrinking. The error is given by the frequency divided by the square-root of the number of events [43] . The average microtubule length was calculated as the average of all instantaneous lengths, where the error represents the s.d. All the values in Supplementary Table 1 represent the average±s.d. for each parameter, from three to five experiments performed under identical conditions. Analysis of microtubule and actin-bundle interactions In a similar fashion to how microtubule–microtubule encounters have been classified in models of cortical microtubule arrays in plants [28] , the interactions between a growing microtubule and an actin bundle were classified into four categories: cross-over, catastrophe, deflection and zippering ( Fig. 2a ). To quantify the probability of these outcomes, the microtubule length L (measured from the plus-end of the microtubule seed to the tip of the microtubule), and the angle θ between the orientation of the tip (defined as the end-most ~2-μm-long section of microtubule) and the actin bundle, were measured at the time of intersection. Thereafter one of the outcomes defined above were assigned by monitoring the subsequent microtubule growth until the next catastrophe. This analysis was performed for n =914 and 708 interactions between growing microtubule plus-ends and F-actin bundles in the presence or absence of 50 nM GFP–TipAct, respectively ( Fig. 2c,e ), and the probability of each outcome calculated as a function of L and θ . For the experiments with variable amounts of GFP–TipAct ( Fig. 2d,g ; Supplementary Fig. 5 ), the analysis was performed only for the encounter angle θ , with the exception that a new interaction outcome was included, namely zipper—snap-off. This analysis was performed for n =459, 421 and 443 interactions for each of the following conditions: 6.25, 12.5 and 25 nM GFP–TipAct, respectively. Analysis of microtubule and actin-bundle array orientation To determine the orientation distributions for the linear arrays of actin bundles and the corresponding microtubule arrays, pixel-by-pixel orientation values were extracted from the fluorescence image files [33] using the Orientation J plugin [44] developed for ImageJ [42] . Among other things, this plugin returns two matrices with the same size as the input image, whose values at each pixel correspond to: (1) orientation (in radians, from— π /2 to π /2), and (2) coherency, which indicates the degree of co-alignment of a given pixel relative to its neighbours within a user-defined window (set to vary from 0 for no co-alignment, to 1 for full co-alignment). In all cases, we used the Gaussian gradient analysis method in Orientation J [44] with a window size of three pixels. Histograms of microtubule and actin bundle orientation angle, θ MT and θ ACTIN , were constructed using the values of the orientation matrix weighted by the coherency, all with a bin size of π /100. This analysis was performed for every frame in fluorescence image stacks that corresponded to 5–10 min of microtubule growth. These histograms were averaged over 2 min of microtubule growth (60 frames), and with these average curves the time evolution of the distribution of θ MT and the average distribution of θ ACTIN were built ( Fig. 3c ). Time zero was defined as the point when the first stack of fluorescence images was recorded, which was typically ~2–3 min after the microtubule polymerization mix was added to the flow cell channel. The same microtubule orientation histograms were used to build the average orientation distribution for all microtubule alignment experiments, both with and without GFP–TipAct, for the cases where the average microtubule length was short (〈 L MT 〉≤19 μm) and long (〈 L MT 〉>19 μm), as defined in Fig. 3d . To this end, all the orientation histograms corresponding to short and long microtubules were collected and shifted along the x axis such that their corresponding mean actin orientation angle (〈 θ ACTIN 〉 ) would fall at 0°. Thereafter, the curves were averaged and the resulting histogram was fit with the Curve Fitting Toolbox of MATLAB using the non-linear least squares method to a Gaussian function of the form: where, A is a constant, μ the mean location, σ the s.d. and B an offset due to noise. The value of μ represents the difference in mean orientation between the microtubules and the actin bundle array, that is, 〈 θ ACTIN 〉 — θ MT , which can be understood as the ‘centering efficiency’, the smaller its value, the better the actin–microtubule co-alignment. On the other hand, the value of σ can be interpreted as the ‘focusing efficiency’, that is, the smaller its value, the more globally the microtubule array has been aligned by the underlying actin bundle array. We performed this for n =6 experiments with GFP–TipAct comprising n =17 histograms for long microtubules and 18 histograms for short microtubules, and for n =9 experiments without GFP–TipAct comprising 9 histograms for long microtubules and 11 histograms for short microtubules. How to cite this article: Preciado López, M. et al. Actin–microtubule coordination at growing microtubule ends. Nat. Commun. 5:4778 doi: 10.1038/ncomms5778 (2014).